The phosphatase JKAP/DUSP22 inhibits T-cell receptor signalling and autoimmunity by inactivating Lck JNK pathway-associated phosphatase (JKAP, also known as DUSP22 or JSP-1) is a JNK activator. The in vivo role of JKAP in immune regulation remains unclear. Here we report that JKAP directly inactivates Lck by dephosphorylating tyrosine-394 residue during T-cell receptor (TCR) signalling. JKAP-knockout T cells display enhanced cell proliferation and cytokine production. JKAP-knockout mice show enhanced T-cell-mediated immune responses and are more susceptible to experimental autoimmune encephalomyelitis (EAE). In addition, the recipient mice that are adoptively transferred with JKAP-knockout T cells show exacerbated EAE symptoms. Aged JKAP-knockout mice spontaneously develop inflammation and autoimmunity. Thus, our results indicate that JKAP is an important phosphatase that inactivates Lck in the TCR signalling turn-off stage, leading to suppression of T-cell-mediated immunity and autoimmunity. T cells play a central role in the adaptive immune response and in autoimmunity. T-cell activation is triggered by T-cell receptor (TCR) signalling. Having accurate and well-controlled TCR signalling machinery is essential for the adaptive immune response. Following antigen recognition, engagement of TCR complexes leads to a signalling cascade of protein tyrosine kinases and adaptors. Phosphorylation and activation of Lck, a Src-family tyrosine kinase, is an early and critical step in pre-TCR and TCR signalling. The activated Lck phosphorylates immunoreceptor tyrosine-based activation motifs of the ζ chain that subsequently recruits and activates the tyrosine kinase ZAP-70, leading to the activation of downstream MAPKs and NF-κB [1] . Mice with Lck deficiency show a partial block of T-cell development and defective TCR signalling in both thymocytes and peripheral T cells [2] . Lck kinase activity is tightly controlled by conformational changes induced by phosphorylation and dephosphorylation of two critical tyrosine residues, Y394 and Y505 (refs 3 , 4 , 5 ). Lck Y505 phosphorylation by CSK tyrosine kinase induces a closed and inactive conformation of Lck, whereas CD45-mediated dephosphorylation of Y505 stimulates an open and active conformation of Lck [6] , [7] . Furthermore, trans-autophosphorylation of Lck at Y394 promotes optimal Lck activation [4] . Through the use of individual phosphatase knockout mice, several protein tyrosine phosphatases (PTPs)—including CD45 (Ptprc), SHP-1 (PTP1C, PTPN6), PTPN22 (PEP, LYP), PTP-PEST (PTPN12) and TCPTP (PTPN2)—have been shown to attenuate T-cell activation [1] , [8] , [9] . However, SHP-1 is not essential for the inhibition of TCR signalling using T-cell-conditional SHP-1 knockout mice [10] . To date, the physiological phosphatase that directly dephosphorylates Lck at Y394 to turn off TCR signalling remains elusive. JNK pathway-associated phosphatase (JKAP, also known as DUSP22 or JSP-1) is a novel dual-specificity phosphatase that specifically activates the kinase JNK [11] , [12] . Overexpression of JKAP selectively activates JNK [11] , [13] , whereas JKAP-knockout murine embryonic fibroblasts lack JNK activation in response to stimulation by TNF-α or TGF-β [11] . JKAP regulates not only the JNK pathway but also various substrates in other signalling cascades. JKAP suppresses IL-6-induced STAT3 activation [14] . Serine-118 of oestrogen receptor-α is dephosphorylated by JKAP, which in turn attenuates oestrogen-mediated signalling in breast cancer cells [15] . JKAP also acts as a tyrosine phosphatase to dephosphorylate and inactivate focal adhesion kinase, leading to the suppression of cell motility [16] . However, the physiological role of JKAP in TCR signalling and immune regulation remains unknown. Here we report that JKAP downregulates the TCR-induced T-cell activation through direct dephosphorylation and inactivation of Lck at Y394, leading to the suppression of T-cell immune responses and autoimmunity. Enhanced TCR signalling in JKAP-knockout T cells To examine the in vivo role of JKAP in T cells, we have generated JKAP-knockout mice by gene-targeting ( Supplementary Fig. 1a ) [11] . The expression of JKAP was detectable in murine wild-type but not JKAP-knockout splenic T cells ( Supplementary Fig. 1b–d ). T-cell development was normal in JKAP-knockout mice ( Supplementary Fig. 2 ). Development of thymus-derived T regulatory cells (Treg) and the function of spleen-derived Treg were unaffected by JKAP deficiency ( Supplementary Fig. 3 ). To determine whether JKAP regulates T-cell activation, we isolated primary T cells from wild-type and JKAP-knockout mice and induced T-cell activation by anti-CD3 with or without anti-CD28 costimulation. The expression levels of T-cell activation markers CD69 and CD25 were similar in unstimulated wild-type and JKAP-knockout T cells ( Fig. 1a ). On anti-CD3 stimulation, these levels of T-cell activation markers in JKAP-knockout T cells were higher than those in wild-type T cells ( Fig. 1a and Supplementary Fig. 4a,b ). Furthermore, JKAP-knockout T cells underwent more cell divisions ( Fig. 1b ) and displayed enhanced anti-CD3-induced calcium flux responses ( Supplementary Fig. 4c ). JKAP-knockout T cells produced more interleukine-2 (IL-2) and interferon-γ (IFN-γ) than those of wild-type T cells, whereas IL-4 production was much lower in both wild-type and JKAP-knockout T cells on TCR signalling ( Fig. 1c and Supplementary Fig. 5 ). Both JKAP-knockout CD4 + and CD8 + T cells exhibited increased T-cell proliferation, activation and IFN-γ production on anti-CD3 stimulation ( Supplementary Fig. 6 ). JKAP-knockout CD4 + T cells also showed increased IL-2 production on TCR signalling ( Supplementary Fig. 6e ). These data indicate that JKAP-knockout T cells are intrinsically hyper-responsive to TCR signalling. 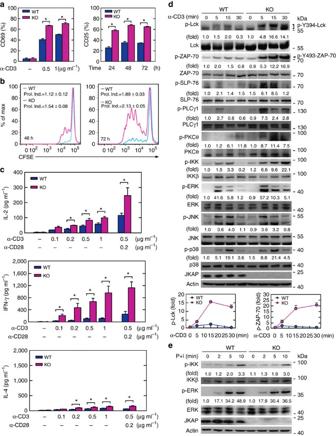Figure 1: JKAP deficiency enhances T-cell activation and TCR signalling. (a) Flow cytometry analyses of T-cell activation markers CD69 (0–1 μg ml−1, 12 h; left panel) and CD25 (0.5 μg ml−1, 24–72 h; right panel) on murine splenic T cells on anti-CD3 stimulation. (b) Carboxyfluorescein diacetate succinimidyl diester dilution assays of T-cell proliferation at 48 h (left panel) and 72 h (right panel) on anti-CD3 (0.5 μg ml−1) stimulation. (c) ELISAs of IL-2, IFN-γ and IL-4 levels in culture supernatants from splenic T cells treated with anti-CD3 (0–1 μg ml−1) stimulation or anti-CD3 (0.5 μg ml−1) plus anti-CD28 (0.2 μg ml−1) costimulation for 24 h. (d) Immunoblotting of various TCR signaling molecules in purified splenic T cells on anti-CD3 (5 μg ml−1) stimulation. (e) Immunoblotting of the phosphorylation of IKK and ERK in splenic T cells on phorbol myristate acetate plus ionomycin (P+I) treatment. Relative fold changes were normalized to total protein levels and are shown at the bottom of the panel (d,e). Quantification of p-Lck (Y394) and p-ZAP-70 (Y493) levels is shown at the bottom of the panel (d). Data are presented as means±s.d. Two-tailed Student’st-test, *P<0.05. Data are representative of at least three independent experiments. Prol. Ind., proliferation index; WT, wild-type; KO, JKAP-knockout. Figure 1: JKAP deficiency enhances T-cell activation and TCR signalling. ( a ) Flow cytometry analyses of T-cell activation markers CD69 (0–1 μg ml −1 , 12 h; left panel) and CD25 (0.5 μg ml −1 , 24–72 h; right panel) on murine splenic T cells on anti-CD3 stimulation. ( b ) Carboxyfluorescein diacetate succinimidyl diester dilution assays of T-cell proliferation at 48 h (left panel) and 72 h (right panel) on anti-CD3 (0.5 μg ml −1 ) stimulation. ( c ) ELISAs of IL-2, IFN-γ and IL-4 levels in culture supernatants from splenic T cells treated with anti-CD3 (0–1 μg ml −1 ) stimulation or anti-CD3 (0.5 μg ml −1 ) plus anti-CD28 (0.2 μg ml −1 ) costimulation for 24 h. ( d ) Immunoblotting of various TCR signaling molecules in purified splenic T cells on anti-CD3 (5 μg ml −1 ) stimulation. ( e ) Immunoblotting of the phosphorylation of IKK and ERK in splenic T cells on phorbol myristate acetate plus ionomycin (P+I) treatment. Relative fold changes were normalized to total protein levels and are shown at the bottom of the panel ( d , e ). Quantification of p-Lck (Y394) and p-ZAP-70 (Y493) levels is shown at the bottom of the panel ( d ). Data are presented as means±s.d. Two-tailed Student’s t -test, * P <0.05. Data are representative of at least three independent experiments. Prol. Ind., proliferation index; WT, wild-type; KO, JKAP-knockout. Full size image We further dissected the effect of JKAP on the regulation of TCR signalling. The tyrosine phosphorylation levels of TCR proximal signalling molecules, such as Lck and ZAP-70, were enhanced in anti-CD3-stimulated JKAP-knockout T cells, preceding the induction of TCR distal signalling proteins, including ERK and IKK ( Fig. 1d ). Furthermore, on anti-CD3 plus anti-CD4 costimulation, the phospho-Y394-Lck levels peaked at 2 min and 0.5 min in wild-type and JKAP-knockout T cells, respectively ( Supplementary Fig. 7a ). The phospho-Y394-Lck levels in JKAP-knockout T cells were more sustained than those in wild-type T cells after anti-CD3 stimulation ( Supplementary Fig. 7b ). These data indicate that loss of JKAP efficiently induces sustained phospho-Y394-Lck levels on TCR signalling. In contrast, JKAP deficiency did not disturb the activation of ERK and IKK induced by phorbol myristate acetate plus ionomycin stimulation, which bypasses TCR proximal signalling ( Fig. 1e ). These data suggest that JKAP targets an upstream regulator of TCR signalling but does not directly dephosphorylate ERK or IKK. The inhibitory role of JKAP in TCR signalling was further verified in Jurkat T cells by JKAP overexpression and shRNA knockdown approaches ( Supplementary Fig. 8 ). Taken together, JKAP deficiency results in enhanced TCR signalling, which in turn promotes T-cell activation, proliferation and cytokine secretion. JKAP directly inactivates Lck on TCR signalling We found that JKAP suppressed proximal TCR signalling and that Lck was the most upstream protein among the signalling molecules affected in JKAP-knockout T cells ( Fig. 1d ); thus, we asked whether JKAP targets Lck on anti-CD3 stimulation. JKAP interacted with Lck in unstimulated murine primary T cells; this interaction was further induced on anti-CD3 stimulation ( Fig. 2a ). In contrast, JKAP did not interact with Fyn, a Src-family tyrosine kinase, in murine splenic T cells ( Fig. 2a ). The JKAP/Lck interaction was also detected in co-transfected HEK293T cells; this interaction was further enhanced on treatment with sodium pervanadate, a tyrosine phosphatase inhibitor ( Supplementary Fig. 9a,b ), suggesting that tyrosine phosphorylation enhances the JKAP/Lck interaction. Moreover, the JKAP/Lck interaction was also enhanced using the catalytically inactive JKAP-C88S mutant ( Supplementary Fig. 9c ). JKAP co-localized with Lck at the cell membrane in the transfected HEK293T cells ( Supplementary Fig. 9d ), and in the anti-CD3-stimulated Jurkat T cells ( Fig. 2b ). Direct interaction between JKAP and Lck was confirmed using purified GST-JKAP and Flag-Lck proteins ( Fig. 2c ). The interaction between JKAP and Lck, but not between JKAP and ZAP-70, was also detected using AlphaScreen analysis ( Supplementary Fig. 10 ), which is a bead-based proximity assay for examining protein–protein interaction in a constrained distance (~200 nm) [17] . We further showed that JKAP directly interacted with Lck, but not PKCθ, in Jurkat T cells using fluorescence resonance energy transfer (FRET) analysis ( Fig. 2d ), which can detect an intra- or inter-molecular interaction within nanometer-scale apposition [18] . The normalized FRET efficiencies were 6.9±4.2%, 5.3±2.9%, 25.3±5.1% and 8.9±3.2% in cells co-expressing CFP plus YFP, CFP plus YFP-Lck, CFP-JKAP plus YFP-Lck and CFP-JKAP plus YFP-PKCθ, respectively ( Fig. 2d ). Collectively, these data indicate that Lck is the direct substrate of JKAP in TCR signalling. 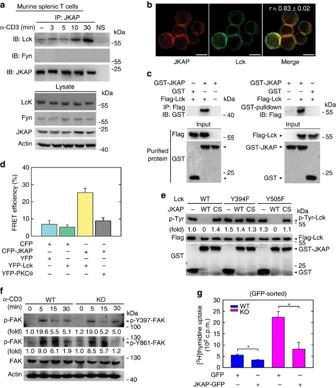Figure 2: JKAP directly interacts with and dephosphorylates Lck. (a) Immunoprecipitation with anti-JKAP and then immunoblotting with anti-Lck of lysates from murine splenic T cells. NS, normal serum. (b) Confocal microscope analysis of JKAP and Lck in stimulated with anti-CD3 (5 μg ml−1, 5 min) and then subjected to double immunostaining with Atto565-congugated anti-JKAP antibody (red) and anti-Lck antibody (green).r, Pearson’s correlation coefficients (mean±s.e.m.) are shown. Scale bar, 10 μm. (c)In vitrobinding assays of purified Flag-Lck and GST-JKAP or GST proteins. Left, anti-Flag immunoprecipitation; right, GST-pulldown. (d) FRET analysis of the direct interaction between CFP-JKAP and YFP-Lck in live Jurkat T cells. (e)In vitrophosphatase reactions of JKAP using purified Flag-Lck WT, Y394F or Y505F proteins as the substrates. CS, the catalytically inactive JKAP-C88S mutant. (f) Immunoblotting of p-FAK (Y397) and p-FAK (Y861) in murine splenic T cells on anti-CD3 (5 μg ml−1) stimulation. Relative fold changes were normalized to total FAK protein levels and are shown at the bottom of each panel. (g) [3H]thymidine incorporation assays in GFP+-T cells that were sorted from murine splenic T cells transfected with empty vector (pCMV6-GFP) or ectopic GFP-JKAP. Data are presented as means±s.d. Two-tailed Student’st-test, *P<0.05. Data are representative of four independent experiments. WT, wild-type; KO, JKAP-knockout. Figure 2: JKAP directly interacts with and dephosphorylates Lck. ( a ) Immunoprecipitation with anti-JKAP and then immunoblotting with anti-Lck of lysates from murine splenic T cells. NS, normal serum. ( b ) Confocal microscope analysis of JKAP and Lck in stimulated with anti-CD3 (5 μg ml −1 , 5 min) and then subjected to double immunostaining with Atto565-congugated anti-JKAP antibody (red) and anti-Lck antibody (green). r , Pearson’s correlation coefficients (mean±s.e.m.) are shown. Scale bar, 10 μm. ( c ) In vitro binding assays of purified Flag-Lck and GST-JKAP or GST proteins. Left, anti-Flag immunoprecipitation; right, GST-pulldown. ( d ) FRET analysis of the direct interaction between CFP-JKAP and YFP-Lck in live Jurkat T cells. ( e ) In vitro phosphatase reactions of JKAP using purified Flag-Lck WT, Y394F or Y505F proteins as the substrates. CS, the catalytically inactive JKAP-C88S mutant. ( f ) Immunoblotting of p-FAK (Y397) and p-FAK (Y861) in murine splenic T cells on anti-CD3 (5 μg ml −1 ) stimulation. Relative fold changes were normalized to total FAK protein levels and are shown at the bottom of each panel. ( g ) [ 3 H]thymidine incorporation assays in GFP + -T cells that were sorted from murine splenic T cells transfected with empty vector (pCMV6-GFP) or ectopic GFP-JKAP. Data are presented as means±s.d. Two-tailed Student’s t -test, * P <0.05. Data are representative of four independent experiments. WT, wild-type; KO, JKAP-knockout. Full size image The inhibitory phosphorylation site Y505 and the activated phosphorylation site Y394 are two critical phosphorylation sites that regulate Lck kinase activity [1] . Next, we examined which tyrosine residue of Lck is regulated by JKAP. Lck-Y394F and Lck-Y505F mutants were used as the substrates; Lck-Y394F is constitutively autophosphorylated at Y505, whereas Lck-Y505F is constitutively autophosphorylated at Y394 when overexpressed [19] . GST-JKAP-WT but not GST-JKAP-C88S mutant efficiently dephosphorylated Lck-Y505F but not Lck-Y394F ( Fig. 2e ), indicating that Lck Y394 phosphorylation is dephosphorylated by JKAP phosphatase activity. In addition, JKAP can dephosphorylate FAK in an overexpression system [16] , and FAK may associate with Lck in anti-CD3-stimulated T-cell clones [20] ; therefore, we asked whether JKAP also dephosphorylates FAK in T cells. The FAK phosphorylation level was not enhanced in JKAP-knockout T cells on anti-CD3 stimulation ( Fig. 2f ), supporting the idea that JKAP deficiency directly upregulates Lck Y394 phosphorylation during TCR signalling. Furthermore, the JKAP deficiency-enhanced cell proliferation was blocked by ectopically expressed JKAP on anti-CD3 stimulation ( Fig. 2g ). The data suggest that JKAP directly dephosphorylates and inactivates Lck at Y394 in TCR signalling, which in turn shuts off T-cell activation. Enhanced T-cell immune responses in JKAP-knockout mice Because JKAP suppressed anti-CD3-induced T-cell activation ( Fig. 1 ), we next investigated the in vivo role of JKAP in T-cell-dependent immune responses. Keyhole limpet haemocyanin (KLH)-immunized JKAP-knockout mice, but not KLH-unimmunized JKAP-knockout mice, showed higher serum IFN-γ and IL-17 levels than immunized wild-type mice ( Fig. 3a ). To further examine the activation of JKAP-knockout T cells in response to antigen-specific stimulation, draining lymph nodes were isolated from KLH-immunized mice and restimulated with KLH. JKAP-knockout T cells produced more IFN-γ, IL-17 and IL-4 and showed enhanced proliferation on KLH restimulation ( Fig. 3b,c ), supporting the idea that JKAP deficiency indeed enhances T-cell activation and T-cell function in vivo . Paradoxically, despite increased production of T-cell cytokines in JKAP-knockout mice, the T-cell-dependent antibody production in the serum of JKAP-knockout mice was moderately reduced after primary and secondary immunization ( Fig. 3d,e ). 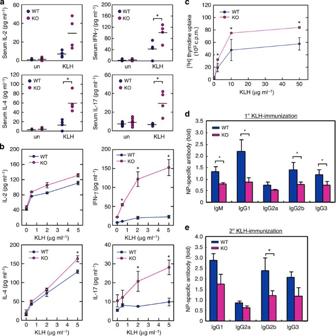Figure 3: Enhanced T-cell-mediated immune responses in JKAP-knockout mice. (a) ELISAs of serum IL-2, IFN-γ, IL-4 and IL-17 levels in unimmunized (un) or at day 7 in KLH-immunized (KLH) JKAP-knockout mice and their wild-type littermates in B6 background (F5). WT,n=4; KO,n=4. (b,c) ELISAs (b) and [3H]thymidine incorporation assay (c) of T cells from draining lymph nodes of KLH-immunized mice at day 7 on restimulation with KLH for 48 and 72 h, respectively. (d,e) ELISAs of nitrophenol-KLH-specific antibody (NP-specific antibody) production in the sera of mice at 14 days after primary immunization (d) or 7 days after secondary immunization (e); results are presented relative to those of the serum from a KLH-immunized wild-type mouse. Data are presented as means±s.d. Two-tailed Student’st-test, *P<0.05. Data are representative of three independent experiments. WT, wild-type; KO, JKAP-knockout. Figure 3: Enhanced T-cell-mediated immune responses in JKAP-knockout mice. ( a ) ELISAs of serum IL-2, IFN-γ, IL-4 and IL-17 levels in unimmunized (un) or at day 7 in KLH-immunized (KLH) JKAP-knockout mice and their wild-type littermates in B6 background (F5). WT, n =4; KO, n =4. ( b , c ) ELISAs ( b ) and [ 3 H]thymidine incorporation assay ( c ) of T cells from draining lymph nodes of KLH-immunized mice at day 7 on restimulation with KLH for 48 and 72 h, respectively. ( d , e ) ELISAs of nitrophenol-KLH-specific antibody (NP-specific antibody) production in the sera of mice at 14 days after primary immunization ( d ) or 7 days after secondary immunization ( e ); results are presented relative to those of the serum from a KLH-immunized wild-type mouse. Data are presented as means±s.d. Two-tailed Student’s t -test, * P <0.05. Data are representative of three independent experiments. WT, wild-type; KO, JKAP-knockout. Full size image We next examined the role of JKAP in B cells. B-cell development was normal in JKAP-knockout mice ( Supplementary Fig. 11 ). JKAP-knockout B cells showed decreased cell activation and proliferation on anti-IgM stimulation ( Fig. 4a,b ). Lyn tyrosine phosphorylation was immediately induced after B-cell receptor (BCR) ligation; the Lyn phosphorylation levels were comparable in wild-type and JKAP-knockout B cells on anti-IgM stimulation ( Fig. 4c ). However, JKAP-knockout B cells showed decreased activation of Syk, ERK and IKK ( Fig. 4d ). Furthermore, we examined antibody production from B cells by immunizing mice with a T-cell-independent antigen, Ficoll. Consistent with the reduced BCR signalling of JKAP-knockout B cells, both IgM and IgG3 levels were decreased in Ficoll-immunized JKAP-knockout mice ( Fig. 4e ). These data indicate that JKAP has an intrinsic role in suppressing TCR signalling and T-cell functions, whereas it plays a positive role in BCR signalling and B-cell function. 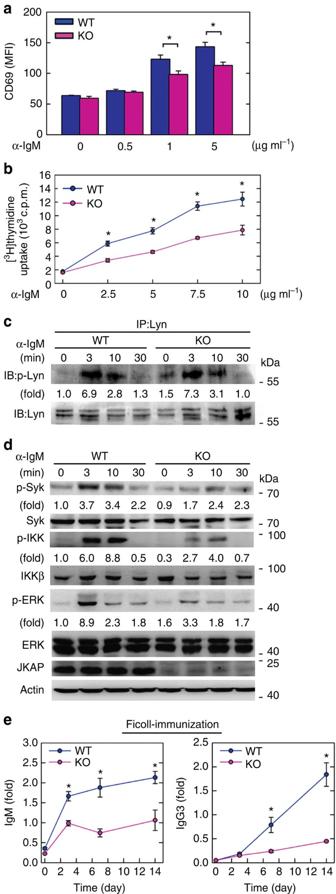Figure 4: Reduced B-cell-mediated immune responses in JKAP-knockout mice. (a) Flow cytometry analyses of CD69 levels on splenic B cells on stimulation with anti-IgM (0–5 μg ml−1) for 24 h. (b) [3H]thymidine incorporation assays of splenic B cells stimulated with anti-IgM for 72 h. (c) Immunoprecipitation with anti-Lyn and then immunoblotting with anti-p-SFK/p-Lyn (Y397) of lysates from splenic B cells on anti-IgM stimulation. (d) Immunoblotting of various BCR signalling molecules in splenic B cells on anti-IgM (10 μg ml−1) stimulation. Relative fold changes were normalized to total protein levels and are shown at the bottom of each blot (c,d). (e) ELISAs of nitrophenol-Ficoll-specific antibodies, IgM and IgG3. WT,n=6; KO,n=6. Data are presented as means±s.d. Two-tailed Student’st-test, *P<0.05. Data are representative of three independent experiments. WT, wild-type; KO, JKAP-knockout. Figure 4: Reduced B-cell-mediated immune responses in JKAP-knockout mice. ( a ) Flow cytometry analyses of CD69 levels on splenic B cells on stimulation with anti-IgM (0–5 μg ml −1 ) for 24 h. ( b ) [ 3 H]thymidine incorporation assays of splenic B cells stimulated with anti-IgM for 72 h. ( c ) Immunoprecipitation with anti-Lyn and then immunoblotting with anti-p-SFK/p-Lyn (Y397) of lysates from splenic B cells on anti-IgM stimulation. ( d ) Immunoblotting of various BCR signalling molecules in splenic B cells on anti-IgM (10 μg ml −1 ) stimulation. Relative fold changes were normalized to total protein levels and are shown at the bottom of each blot ( c , d ). ( e ) ELISAs of nitrophenol-Ficoll-specific antibodies, IgM and IgG3. WT, n =6; KO, n =6. Data are presented as means±s.d. Two-tailed Student’s t -test, * P <0.05. Data are representative of three independent experiments. WT, wild-type; KO, JKAP-knockout. Full size image Exacerbated autoimmunity in JKAP-knockout mice Uncontrolled immune responses, including altered T-cell activation and Th1–Th17 polarization, may lead to autoimmunity. To investigate whether JKAP-knockout mice are more susceptible to autoimmune diseases, mice were immunized with myelin oligodendrocyte glycoprotein (MOG) peptides to induce experimental autoimmune encephalomyelitis (EAE). JKAP-knockout mice developed faster and more severe EAE symptoms compared with those of wild-type mice ( Fig. 5a ). Furthermore, the levels of the proinflammatory cytokines IFN-γ and IL-17 in the sera ( Fig. 5b ), as well as the percentages of phospho-Y394-Lck-positive T cells in the peripheral blood ( Fig. 5c and Supplementary Fig. 12 ), were increased in diseased JKAP-knockout mice. In brain tissues, greater numbers of infiltrating CD4 + T cells were detected in diseased JKAP-knockout mice, whereas similar numbers of infiltrating MAC-1 + cells were detected in diseased wild-type and JKAP-knockout mice ( Fig. 5d ). Infiltrating IFN-γ + Th1 cells and IL-17 + Th17 cells in the brain and the spinal cord were increased in diseased JKAP-knockout mice ( Fig. 5e–g ). The data demonstrate that JKAP-knockout mice were more susceptible to the EAE induction. 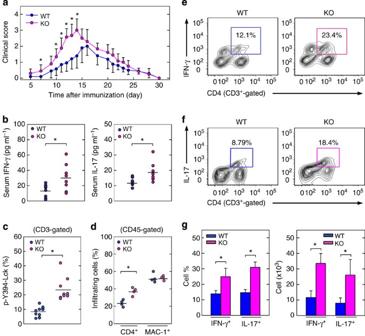Figure 5: Exacerbated EAE in JKAP-knockout mice. (a) The EAE induction in JKAP-knockout mice and their wild-type littermates in B6 background (F5). Disease clinical scores (1–5) of mice are shown. WT,n=15; KO,n=15. (b) ELISAs of serum cytokine levels of EAE-diseased mice at day 14. (c) Flow cytometry analyses of phospho-Y394-Lck levels in peripheral blood T cells from EAE-diseased mice at day 14. (d–f) Flow cytometry analyses of infiltrating CD4+and MAC-1+(d), IFN-γ-producing CD4+cells (CD3+-gated) (e), and IL-17-producing CD4+cells (CD3+-gated) (f) from the brains and spinal cords of MOG-immunized mice at day 14. (g) The percentages and numbers of the cell population in (e,f) were analysed. Five mice were analysed for each group. Data are presented as means±s.d. Kruskal–Wallis test, *P<0.05. Data are representative of at least three independent experiments. WT, wild-type; KO, JKAP-knockout. Figure 5: Exacerbated EAE in JKAP-knockout mice. ( a ) The EAE induction in JKAP-knockout mice and their wild-type littermates in B6 background (F5). Disease clinical scores (1–5) of mice are shown. WT, n =15; KO, n =15. ( b ) ELISAs of serum cytokine levels of EAE-diseased mice at day 14. ( c ) Flow cytometry analyses of phospho-Y394-Lck levels in peripheral blood T cells from EAE-diseased mice at day 14. ( d – f ) Flow cytometry analyses of infiltrating CD4 + and MAC-1 + ( d ), IFN-γ-producing CD4 + cells (CD3 + -gated) ( e ), and IL-17-producing CD4 + cells (CD3 + -gated) ( f ) from the brains and spinal cords of MOG-immunized mice at day 14. ( g ) The percentages and numbers of the cell population in ( e , f ) were analysed. Five mice were analysed for each group. Data are presented as means±s.d. Kruskal–Wallis test, * P <0.05. Data are representative of at least three independent experiments. WT, wild-type; KO, JKAP-knockout. Full size image JKAP deficiency-enhanced EAE is T-cell intrinsic To confirm that the exacerbated EAE symptom in JKAP-knockout mice is caused by the T-cell-intrinsic defect, we adoptively transferred CD4 + T cells from JKAP-knockout or wild-type mice into the irradiated recipient mice and subsequently induced EAE in the recipient mice. The recipient mice that were transferred with JKAP-knockout CD4 + T cells developed more severe EAE symptoms than the control mice ( Fig. 6a ). Consistently, the serum levels of IFN-γ and IL-17 were increased in the diseased recipient mice that were transferred with JKAP-knockout CD4 + T cells ( Fig. 6b ). In addition, the recipient mice that were passively transferred with the encephalitogenic CD4 + T cells from EAE-diseased JKAP-knockout mice were more susceptible to EAE induction than the control mice ( Supplementary Fig. 13 ). These data indicate that JKAP deficiency-mediated pathogenesis of autoimmunity is a T-cell-intrinsic effect. To further examine the function of MOG-specific T cells, splenic T cells were isolated from diseased wild-type and JKAP-knockout mice, and restimulated with MOG peptides; T-cell proliferation and cytokine production were then measured. JKAP-knockout splenic T cells showed enhanced proliferation in response to MOG restimulation ( Fig. 6c ). As expected, MOG-restimulated JKAP-knockout T cells also produced more IL-2, IFN-γ and IL-17 ( Fig. 6c ). However, without additional experiments (such as the bone marrow chimera), we cannot rule out the possibility that the wild-type or JKAP-knockout T cells may not be functionally equivalent. These results suggest that the increased MOG-specific proinflammatory T cells contribute to exacerbated EAE clinical symptoms in JKAP-knockout mice. 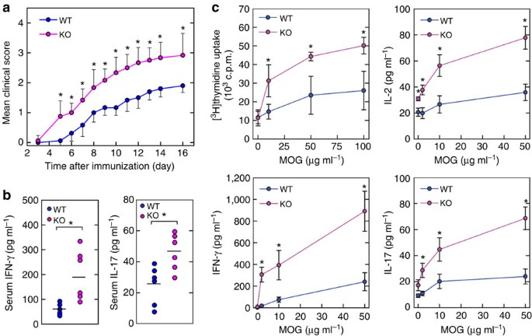Figure 6: JKAP deficiency-enhanced EAE is T-cell intrinsic. (a) The recipient mice were adoptively transferred with CD4+T cells from JKAP-knockout and wild-type mice and then subjected to EAE induction. Disease clinical scores (1–5) of mice are shown. WT,n=8; KO,n=8. (b) ELISAs of serum cytokine levels of EAE-diseased mice at day 14. (c) [3H]thymidine incorporation assays and ELISAs of the splenic T cells obtained from MOG-immunized mice at day 14 on restimulation with MOG peptides for 72 and 48 h, respectively. Data are presented as means±s.d. Kruskal–Wallis test, *P<0.05. Data are representative of two (a,b) or four (c) independent experiments. WT, wild-type; KO, JKAP-knockout. Figure 6: JKAP deficiency-enhanced EAE is T-cell intrinsic. ( a ) The recipient mice were adoptively transferred with CD4 + T cells from JKAP-knockout and wild-type mice and then subjected to EAE induction. Disease clinical scores (1–5) of mice are shown. WT, n =8; KO, n =8. ( b ) ELISAs of serum cytokine levels of EAE-diseased mice at day 14. ( c ) [ 3 H]thymidine incorporation assays and ELISAs of the splenic T cells obtained from MOG-immunized mice at day 14 on restimulation with MOG peptides for 72 and 48 h, respectively. Data are presented as means±s.d. Kruskal–Wallis test, * P <0.05. Data are representative of two ( a , b ) or four ( c ) independent experiments. WT, wild-type; KO, JKAP-knockout. Full size image Inflammation and autoimmunity in aged JKAP-knockout mice One possible consequence of JKAP deficiency-induced T-cell activation on TCR signalling could be the development of autoimmunity and inflammation in aged JKAP-knockout mice. Although gross pathology in young JKAP-knockout mice was unremarkable, serum levels of proinflammatory cytokines, including IFN-γ, IL-17, IL-6 and TNF-α, were significantly elevated in 24-, 48- and 72-week-old JKAP-knockout mice compared with age-matched wild-type littermates ( Fig. 7a ). Higher circulating levels of anti-nuclear antibodies and anti-dsDNA antibodies were detected in sera from aged JKAP-knockout mice ( Fig. 7b ). The percentages of phospho-Y394-Lck-positive T cells in the peripheral blood were also increased in 48- and 72-week-old but not 8-week-old JKAP-knockout mice ( Fig. 7c and Supplementary Fig. 14 ). Splenomegaly was observed in aged JKAP-knockout mice ( Fig. 7d ). Aged JKAP-knockout mice showed the expansion of white pulps in spleens ( Fig. 7e ). Aged JKAP-knockout mice showed the massive infiltration of lymphocytes in liver periportal areas ( Fig. 7f ), lungs ( Fig. 7g ) and renal tubules ( Fig. 7h , upper panel). Kidney tissues from aged JKAP-knockout mice also exhibited the glomerulomegaly with hypersegmentation ( Fig. 7h , lower panel). Conversely, aged wild-type littermates did not develop inflammation and autoimmunity ( Fig. 7d–h ). We further examined and quantified the histological changes of renal tissues. The kidney sections were stained with periodic acid-Schiff (PAS; Fig. 8a ) and Masson’s trichrome ( Fig. 8b ). Glomerular damage, massive mononuclear cell infiltration and tubulointerstitial injury (such as mesangial hypertrophy and glomerular atrophy) were more pronounced in aged JKAP-knockout mice ( Fig. 8c ). These results suggest that aged JKAP-knockout mice develop systemic inflammation and autoimmune diseases. Thus, our results indicate a critical role of JKAP in attenuating T-cell activation through Lck inactivation, leading to downregulation of autoimmune diseases ( Fig. 9 ). 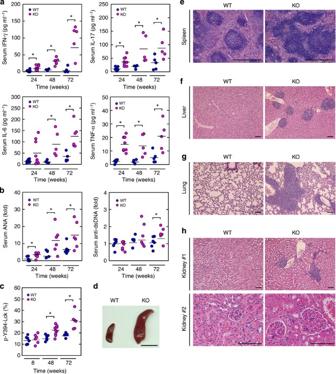Figure 7: Inflammation and autoimmune disorders in aged JKAP-knockout mice. (a,b) ELISAs of serum IFN-γ, IL-17, IL-6 and TNF-α levels (a) and serum anti-nuclear antibodies (ANA) and anti-dsDNA levels (b) in 24-, 48- and 72-week-old JKAP-knockout mice and their wild-type littermates in B6 background (F5).The results of ANA and anti-dsDNA levels are presented relative to those of the sera from their age-matched wild-type mice. WT,n=6; KO,n=6. (c) Flow cytometry analyses of phospho-Y394-Lck levels in peripheral blood T cells from 8-, 48- and 72-week-old JKAP-knockout mice and their wild-type littermates. (d) Splenomegaly observed in 72-week-old JKAP-knockout mice. Scale bar, 1.5 cm. (e–h) Photomicrographs of the spleen (e), the liver (f), the lung (g) and the kidney (h) tissues stained with hematoxylin-eosin. Scale bar, 0.5 mm (e) and 10 μm (f–h). Kruskal–Wallis test, *P<0.05. WT, wild-type; KO, JKAP-knockout. Figure 7: Inflammation and autoimmune disorders in aged JKAP-knockout mice. ( a , b ) ELISAs of serum IFN-γ, IL-17, IL-6 and TNF-α levels ( a ) and serum anti-nuclear antibodies (ANA) and anti-dsDNA levels ( b ) in 24-, 48- and 72-week-old JKAP-knockout mice and their wild-type littermates in B6 background (F5).The results of ANA and anti-dsDNA levels are presented relative to those of the sera from their age-matched wild-type mice. WT, n =6; KO, n =6. ( c ) Flow cytometry analyses of phospho-Y394-Lck levels in peripheral blood T cells from 8-, 48- and 72-week-old JKAP-knockout mice and their wild-type littermates. ( d ) Splenomegaly observed in 72-week-old JKAP-knockout mice. Scale bar, 1.5 cm. ( e – h ) Photomicrographs of the spleen ( e ), the liver ( f ), the lung ( g ) and the kidney ( h ) tissues stained with hematoxylin-eosin. Scale bar, 0.5 mm ( e ) and 10 μm ( f – h ). Kruskal–Wallis test, * P <0.05. WT, wild-type; KO, JKAP-knockout. 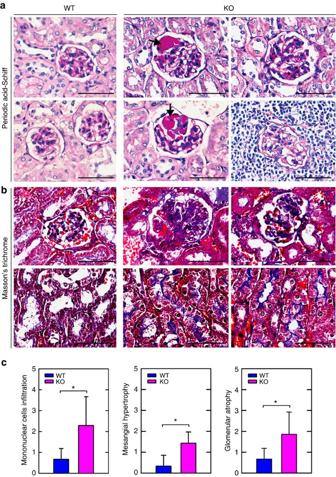Figure 8: Exacerbated renal tissue damage in aged JKAP-knockout mice. (a,b) Representative micrographs of periodic acid-Schiff (PAS)-stained (a) and Masson’s trichrome-stained (b) kidney sections from 72-week-old JKAP-knockout mice and their wild-type littermates in B6 background (F5). Arrows, glomerular sclerosis. Scale bar, 5 μm; original magnification, × 800 (a,b). (c) Quantification of mononuclear cells infiltration, mesangial hypertrophy and glomerular atrophy. WT,n=6; KO,n=7. Data are presented as means±s.d. Kruskal–Wallis test, *P<0.05. WT, wild-type; KO, JKAP-knockout. Full size image Figure 8: Exacerbated renal tissue damage in aged JKAP-knockout mice. ( a , b ) Representative micrographs of periodic acid-Schiff (PAS)-stained ( a ) and Masson’s trichrome-stained ( b ) kidney sections from 72-week-old JKAP-knockout mice and their wild-type littermates in B6 background (F5). Arrows, glomerular sclerosis. Scale bar, 5 μm; original magnification, × 800 ( a , b ). ( c ) Quantification of mononuclear cells infiltration, mesangial hypertrophy and glomerular atrophy. WT, n =6; KO, n =7. Data are presented as means±s.d. Kruskal–Wallis test, * P <0.05. WT, wild-type; KO, JKAP-knockout. 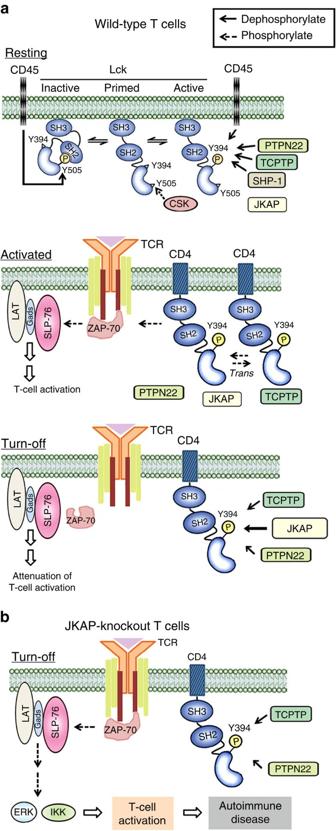Figure 9: The model of JKAP-mediated suppression of T-cell activation and autoimmune diseases through dephosphorylating Lck at Y394. (a) In resting T cells, Lck is dynamically regulated through phosphorylation and dephosphorylation at Y505 and Y394 residues. Phosphorylation of Y505 by CSK causes an inactive conformation; dephosphorylation of phospho-Y505 by CD45 provides the opportunity for trans-autophosphorylation of Lck at Y394, which promotes an active conformation in resting T cells. Several phosphatases, but not including JKAP, participate in the downregulation of phospho-Y394-Lck levels (upper panel), leading to the restriction of the active Lck levels in resting T cells. After TCR ligation, the activated Lck phosphorylates immunoreceptor tyrosine-based activation motifs of the ζ chain, which subsequently recruits and activates ZAP-70, leading to the assembly of proximal SLP-76 signalling complexes and the activation of downstream signalling molecules. JKAP participates in tuning TCR signalling in the activated stage (middle panel). In the TCR signalling turn-off stage, JKAP is the major phosphatase that directly dephosphorylates phospho-Y394-Lck, leading to the attenuation of T-cell activation (lower panel). (b) Loss of JKAP efficiently induces sustained phospho-Y394-Lck levels on TCR signaling, leading to the pathogenesis of autoimmune diseases. Full size image Figure 9: The model of JKAP-mediated suppression of T-cell activation and autoimmune diseases through dephosphorylating Lck at Y394. ( a ) In resting T cells, Lck is dynamically regulated through phosphorylation and dephosphorylation at Y505 and Y394 residues. Phosphorylation of Y505 by CSK causes an inactive conformation; dephosphorylation of phospho-Y505 by CD45 provides the opportunity for trans-autophosphorylation of Lck at Y394, which promotes an active conformation in resting T cells. Several phosphatases, but not including JKAP, participate in the downregulation of phospho-Y394-Lck levels (upper panel), leading to the restriction of the active Lck levels in resting T cells. After TCR ligation, the activated Lck phosphorylates immunoreceptor tyrosine-based activation motifs of the ζ chain, which subsequently recruits and activates ZAP-70, leading to the assembly of proximal SLP-76 signalling complexes and the activation of downstream signalling molecules. JKAP participates in tuning TCR signalling in the activated stage (middle panel). In the TCR signalling turn-off stage, JKAP is the major phosphatase that directly dephosphorylates phospho-Y394-Lck, leading to the attenuation of T-cell activation (lower panel). ( b ) Loss of JKAP efficiently induces sustained phospho-Y394-Lck levels on TCR signaling, leading to the pathogenesis of autoimmune diseases. Full size image Having accurate and well-controlled TCR signalling machinery is essential for the adaptive immune response. Here we unequivocally demonstrate that JKAP is an important phosphatase that directly dephosphorylates Lck at Y394, leading to attenuation of T-cell activation in the TCR signalling turn-off stage. Lck is dynamically regulated through phosphorylation and dephosphorylation of its two tyrosine residues (Y505 and Y394). Phosphorylation of Y505 by CSK causes an inactive, closed conformation, whereas autophosphorylation of Y394 promotes an active, open conformation in resting T cells [1] , [8] , [9] . CD45 can dephosphorylate phospho-Y505-Lck (the inactive Lck); conversely, it can also, albeit less efficiently, dephosphorylate phospho-Y394-Lck (the active Lck) in resting T cells [7] . Dephosphorylation of phospho-Y394-Lck will decrease the levels of active Lck in response to dephosphorylation of phospho-Y505-Lck in resting T cells. Several PTPs, including SHP-1, PTPN22 and TCPTP, also dephosphorylate phospho-Y394-Lck in resting T cells [8] , [9] . We found that the phospho-Y394-Lck-positive T cells were not induced in peripheral blood from 8-week-old JKAP-knockout mice, indicating that JKAP did not play a redundant role in the downregulation of the active Lck levels in resting T cells ( Fig. 9a , upper panel). In addition, we found that JKAP-knockout mice did not have any overt alterations in T-cell development. Similarly, T-cell development is not affected in DUSP4-deficient mice [21] , DUSP14-deficient mice [22] , SHP-1 T-cell-specific conditional knockout mice [10] or T-cell-specific dominant-negative SHP-2 transgenic mice [23] . However, without additional experiments (such as breeding JKAP-knockout mice to a TCR transgenic mouse line), we cannot rule out the possibility that JKAP could participate in the attenuation of thymocyte development. Intriguingly, deletions of PTPN22 and TCPTP have been shown to display augmented thymocyte-positive selection [24] , [25] , implicating that PTPN22 and TCPTP may compensate for JKAP deficiency, leading to normal thymocyte development in JKAP-knockout mice. On TCR engagement, trans-autophosphorylation of Lck at Y394 promotes optimal Lck activation that exceeds the threshold of phospho-Y394-Lck levels, leading to the induction of downstream signalling cascades ( Fig. 9a , middle panel). Following TCR signalling, efficient dephosphorylation of phospho-Y394-Lck attenuates the T-cell activation in the turn-off stage. The roles of other PTPs on the Lck regulation are different in activated T cells. Lck Y394 phosphorylation is not induced in anti-CD3-stimulated CD45-deficient T cells owing to the blocking of TCR signalling [26] . On anti-CD3 stimulation, PTPN22 deficiency enhances Lck Y394 phosphorylation in effector/memory T cells but not in naïve T cells [24] . T-cell-specific depletion of TCPTP increases Lck Y394 phosphorylation mainly in CD8 + but not CD4 + naïve T cells during TCR signalling [25] . Our results show that JKAP directly dephosphorylates Lck at Y394 in the TCR signalling turn-off stage ( Fig. 9a , lower panel); distinct from PTPN22 and TCPTP, JKAP deficiency enhances Lck Y394 hyperphosphorylation in both CD4 + and CD8 + naïve T cells on TCR signalling. Lck hyperactivation leads to an overall enhanced TCR downstream signalling, including JNK activation; however, JNK activation was modestly reduced in JKAP-knockout T cells on anti-CD3 stimulation. JKAP specifically activates JNK in overexpression systems [11] , [13] ; the JKAP deficiency-downregulated JNK activation could be counteracted by the Lck-induced JNK activation on TCR signalling. In addition, anti-CD3-stimulated p38 activation was not affected in JKAP-knockout splenic T cells. Activation of p38 is inhibited by ERK in TGF-β signalling [27] ; it is plausible that anti-CD3-induced p38 activation is offset by ERK activation in JKAP-knockout T cells. JKAP and PTPs share a strikingly similar structure and utilize the same cysteine-based catalytic mechanism. When the critical cysteine residue within a PTP phosphatase domain is mutated, usually to a serine residue, that PTP usually retains the ability to bind to the phosphotyrosyl substrate but cannot execute a nucleophilic attack on its substrate [28] . Indeed, the phosphatase-dead JKAP-C88S mutant proteins exhibited a stronger interaction with Lck compared with JKAP-WT, further supporting that Lck is a JKAP substrate. Our data demonstrate that JKAP plays a negative role in TCR signalling, whereas it positively regulates BCR signalling. Although JKAP-knockout mice showed reduced antibody production on immunization with T-cell-dependent or T-cell-independent antigens, aged JKAP-knockout mice still showed an increase in autoantibody production. Our data suggest that JKAP deficiency in T cells may contribute to the development of autoimmunity; however, we cannot rule out the possibility that JKAP may regulate the autoreactive B-cell populations through different mechanisms such as negative selection and long-term survival [29] . In addition, JKAP may participate in the functions of B cells that suppress autoimmune diseases [30] . As JKAP-knockout B cells showed reduced activation of Syk, JNK, ERK and p38 on anti-IgM stimulation, JKAP may stimulate a Syk-activating kinase or inactivate a Syk-inhibiting kinase on anti-IgM stimulation. JKAP may also inhibit a phosphatase that inhibits Syk or its upstream kinase(s). The study of these possibilities is beyond the scope of this report. Dysregulation of the immune system has been shown to participate in the development of autoimmunity [29] . For example, T cells contribute to the initiation and development of systemic lupus erythematosus [31] . Other abnormalities associated with T-cell functions also contribute to the pathogenesis of autoimmune diseases. For example, lupus T cells are shown to have the genetic/epigenetic aberrations of PTPN22 and STAT4, and the increased levels of CD40 ligand and CD44, as well as mitochondrial dysfunction [29] , [32] , [33] , [34] . Here we show that JKAP dysfunction in T cells also leads to autoimmunity. Treg deficiencies also occur in patients with autoimmune diseases [30] . Although JKAP deficiency did not affect the suppressive function of Treg, we cannot rule out that JKAP may disturb the functions of other types of suppressor cells. In addition, genome-wide association studies have identified a number of genes, including ITGAM and SIAE , associated with autoimmune diseases [34] ; nevertheless, many more genetic risk loci of autoimmune diseases remain to be uncovered. It is important to examine the genetic and epigenetic regulations of JKAP in autoimmune diseases in the future. In conclusion, JKAP plays an important role in the suppression of TCR signalling via directly inactivating Lck, leading to reduced T-cell-mediated immune responses. Thus, loss of JKAP-mediated inhibition in T cells could contribute to the pathogenesis of autoimmune diseases ( Fig. 9b ). Mice JKAP-knockout 129/Ola embryonic stem cells (129/Ola background) were microinjected into C57BL/6 blastocysts to generate chimeric mice [11] . Mice were backcrossed to C57BL/6 background for five generations (F5; ~97%) and F10. The genotype of the offspring was determined by PCR analysis. The data presented in this study were performed on sex-matched, 4–10-week-old littermates. For immunization experiments, 8-week-old sex-matched mice were used. For EAE experiments, 8-week-old female mice were used. For aged mouse studies, 4-week-old sex-matched mice were monitored for 72 weeks. Mice were randomly assigned to in vivo animal experiments. All animal protocols were approved by the Institutional Animal Care and Use Committee of the National Health Research Institutes, Taiwan. Cell lines and transfection Human Jurkat T leukaemia cells (American Type Cell Culture (ATCC): TIB-152) and their variant, J-TAg cells [22] , were cultured in RPMI-1640 medium (Invitrogen) containing 10% fetal calf serum (FCS; Invitrogen) plus penicillin (10 units ml −1 ) and streptomycin (10 μg ml −1 ) (Invitrogen). HEK293T cells (ATCC: CRL-11268) were cultured in Dulbecco’s modified Eagle’s medium (Invitrogen) containing 10% FCS plus penicillin (10 units ml −1 ) and streptomycin (10 μg ml −1 ). The cells were free of mycoplasma contamination. Plasmids were transfected into primary T cells, Jurkat T and J-TAg cells by electroporation method using the Neon transfection system (Invitrogen). Transfection of HEK293T cells was performed using polyethylenimine reagents. Plasmids The expression plasmid for human JKAP was generated using a cDNA pool of H1299 cells as the PCR template; the primers used were 5′-CGCGGATCCATGGGGAATGGGATGAA-3′ and 5′-CGCCTCGATCAGTCTTCTGAGAAAGGCCCAG-3′. The JKAP-C88S mutant expression plasmid was generated by site-directed mutagenesis and confirmed by DNA sequencing [16] . A 19-nucleotide sequence 5′-ACACTGGTGATCGCATACA-3′ (shJKAP), corresponding to human JKAP coding sequence residues 289–307, was used for designing the inverted repeat insertion [16] . A human Lck-encoding fragment was amplified using a cDNA pool of Jurkat T cells as the PCR template; the primers used were 5′-GAGGCGATCGCCACCATGGGCTGTGGCTGCAGCTCA-3′ and 5′-GCGACGCGTAGGCTGAGGCTGGTACTGGCCCTC-3′. The fragment was inserted into pCMV6-AC-DDK (OriGene Technologies). Flag-tagged Lck-Y394F and Y505F mutant-expressing vectors were generated by site-directed mutagenesis and confirmed by DNA sequencing. Antibodies and reagents Anti-phosphotyrosine antibody was from Upstate Biotechnology. Anti-Flag (M2) and anti-β-actin antibodies were from Sigma-Aldrich. Anti-myc monoclonal antibody was prepared from a culture of hybridoma clone 9E10 (ATCC). Stimulatory anti-CD3 (OKT3, 145-2C11 and 500A2) antibodies were from BD Biosciences. The antibodies for flow cytometry—including anti-mCD3ε-FITC (145-2C11), anti-CD45-FITC (30-F11), anti-CD62L (MEL-14), anti-mCD69-FITC (H1.2F3), anti-Foxp3-PE (150D), anti-CD25-PE (PC61), anti-CD44-PE (IM7) and anti-hCD3-PE-Cy7 (HIT3a)—were purchased from BioLegend. Anti-IL-17A-Alexa Fluor 647 (TC11-18H10), anti-mCD3e-APC (145-2C11), anti-mCD4-pacific blue (RM4-5) and anti-CD8-APC-Cy7 (53-6.7) antibodies were purchased from BD Biosciences. All antibodies for flow cytometry were used at 1:20 or 1:50 dilutions. Anti-DUSP22 antibody was from Abnova. Anti-JKAP (JKAP-N), anti-SLP-76, anti-JNK, anti-ERK and anti-p38 antibodies were generated by immunization of rabbits with individual peptides. Anti-p-ERK (T202/Y204) and anti-p-p38 (T180/Y182) antibodies were generated by immunization of rabbits with individual phospho-peptides; specificities of these antibodies were verified. Anti-p-JNK (Y185) and anti-PKCθ antibody were from Epitomics. Anti-p-Lck (Y394)/p-Lyn (Y397)/p-SFK (Y416), anti-Lck, anti-p-ZAP-70 (Y493), anti-ZAP-70, anti-p-Syk (Y352), anti-Syk, anti-p-SLP-76 (Y145), anti-p-PLC-γ1 (Y783), anti-PLC-γ1, anti-p-IKKα (S176)/p-IKKβ (S180), anti-p-FAK (Y397), anti-p-FAK (Y861) and anti-IKK antibodies were purchased from Cell Signaling Technology. Anti-p-PKCθ (T538) antibody was from Upstate Biotechnology. Anti-Lyn antibody was from GeneTex. All primary antibodies for immunoblot were used at 1:500 or 1:1,000 dilutions. Carboxyfluorescein diacetate succinimidyl diester was purchased from Invitrogen. The rest of the chemicals were purchased from Sigma-Aldrich. Immunoprecipitation and in vitro phosphatase assays Cell extracts were incubated with individual antibodies and protein G-agarose beads in lysis buffer (50 mM Tris (pH 8.0), 150 mM NaCl, 1% Triton X-100, 0.5% deoxycholate, 0.1% SDS, 2 μg ml −1 leupeptin, 5 μg ml −1 aprotinin, 1 mM phenylmethylsulphonyl fluoride, 1 mM dithiothreitol and 1 mM Na 3 VO 4 ) with continuous rotation at 4 °C for 3 h. Immunoprecipitates were washed three times with lysis buffer before immunoblotting analyses or in vitro phosphatase assays. For phosphatase assays, immunoprecipitated complexes were washed once with phosphatase buffer (50 mM Tris (pH 7.0), 50 mM Bis-Tris, 100 mM sodium acetate and 10 mM dithiothreitol). The phosphatase reaction was performed at 37 °C for 30 min, terminated by adding SDS sample buffer and heating at 95 °C for 5 min, followed by immunoblotting [35] . Immunoblotting analysis The phosphatase reaction mixtures or cell extracts were fractionated on SDS–polyacrylamide gel electrophoresis and transferred to polyvinylidene difluoride membranes. The membranes were probed, first with individual primary antibodies and then with horseradish peroxidase-conjugated secondary antibody. The horseradish peroxidase substrate reaction was performed using the SuperSignal chemiluminescent reagent, and the chemiluminescent signal was detected by a BioSpectrum 500 imaging system. Full blots are shown in Supplementary Fig. 15 . Enzyme-linked immunosorbent assays The levels of IL-2, IL-4, IFN-γ, IL-17, IL-6 and TNF-α in the sera or cell culture supernatants were analysed by enzyme-linked immunosorbent assays (ELISAs) as described by the manufacturer (eBioscience). The levels of anti-nuclear antibodies and anti-dsDNA antibodies in the sera were analysed by ELISAs as described by the manufacturer (Alpha Diagnostic International). In vitro T-cell stimulation and proliferation Jurkat T-cell stimulation was performed using an anti-CD3 antibody (OKT3, 5 μg ml −1 ) [36] . To purify murine CD3 + T cells, red blood cell-depleted splenocytes were isolated and negatively selected using a cocktail of biotin-conjugated anti-B220, anti-CD11b and anti-CD49b antibodies (Biolegend) on a MACS column (Miltenyi Biotec). Purified splenic T cells were untreated or stimulated with soluble anti-CD3 (145-2C11, 3 μg ml −1 ) or phorbol myristate acetate (0.05 μg ml −1 ) plus ionomycin (1 μg ml −1 ). For T-cell proliferation assays, splenic T cells were stained with carboxyfluorescein diacetate succinimidyl diester and stimulated with soluble anti-CD3 antibody (145-2C11, 3 μg ml −1 ) for 48 or 72 h followed by flow cytometry analysis [21] . Confocal microscope analysis The tested cells were fixed in 4% paraformaldehyde. After permeation with 0.25% Triton X-100, the cells were blocked with 5% bovine serum albumin. Nuclei were detected with 4',6-diamidino-2-phenylindole (Molecular Probes). The coverslides were mounted in mounting medium (Biomeda, USA) and analysed using a Leica TCS SP2 AOBS confocal microscope (Mannheim, Germany). For quantifying colocalization [37] of JKAP with Lck, the Pearson’s correlation coefficient ( r ) was determined using Leica LAS AF software. AlphaScreen analysis for protein–protein interaction AlphaScreen technology was performed according to the manufacturer’s protocol (PerkinElmer, USA). HEK293T cells were co-transfected with Myc-JKAP plus either Flag-Lck or Flag-ZAP-70 for 24 h. The cells were lysed in lysis buffer (20 mM Tris (pH 8.0), 150 mM NaCl, 0.5% NP40, 1 mM EDTA, 2 μg ml −1 leupeptin, 5 μg ml −1 aprotinin, 1 mM phenylmethylsulphonyl fluoride, 1 mM dithiothreitol and 1 mM Na 3 VO 4 ). The cell lysates were incubated with anti-MYC Alpha acceptor beads (PerkinElmer) for 30 min and then incubated with anti-FLAG Alpha donor beads (PerkinElmer) for another 60 min. The Alpha signalling was determined by EnVision 2104 Multilabel Plate Reader (PerkinElmer). FRET assays FRET in live cells was detected using EnVision 2101 Multilabel Plate Reader. The reaction was excited by light passing though a 430-nm filter (with 8 nm bandwidth), and the intensity of emitted fluorescence passing though a 530-nm filter (with 8 nm bandwidth) was recorded. The FRET efficiency was calculated by a ratio method, E =(1− F DA/ F D) × 100%, where F D and F DA are the relative fluorescence intensities of the donor in the absence and presence of the acceptor, respectively. Flow cytometry analysis Thymocytes, splenocytes and lymph node cells from mice were stained with individual fluorochrome-conjugated antibodies as indicated. Cells were harvested, washed with cold PBS buffer, and stained with indicated antibodies for 30 min on ice. For intracellular staining of cytokines and phospho-Y394-Lck, cells were preincubated with Monensin (GolgiStop; BD biosciences), fixed, permeabilized with BD Cytofix/Cytoperm and stained for individual cytokines or phospho-Y394-Lck. Data were acquired with a FACSCanto II (BD Biosciences) and analysed with FlowJo analytical software (TreeStar). Morphological examinations The pathological indexes of kidney specimen are determined by light microscopic examinations (stained with hematoxylin and eosin, PAS, and Masson’s trichrome) [38] . Glomerular sclerosis in 30 glomeruli per mouse was assessed. Tubulointersitial injury was examined based on the percentage of tubules showing dilatation or atrophy in interstitial areas of renal cortex per mouse. Different indexes—including lymphocyte infiltration, mesangial stalk PAS positivity (mesangial hypertrophy), glomerular sclerosis, tubulointerstitial injury and glomerular atrophy—were analysed by using the scoring system as follows; 0, none; 1, ⩽ 10%; 2, 11–25%; 3, 26–45%; 4, 46–75% and 5, >76%. Scoring of all kidney sections was done by a pathologist in a blinded manner. Immunization and induction of EAE To examine the T-cell-mediated humoral immune responses, mice were immunized by intraperitoneal injection of nitrophenol (NP)-coupled keyhole limpet haemocyanin (KLH) emulsified in aluminium hydroxide gel or NP–Ficoll (Biosearch Technologies Inc.) in PBS buffer. The production of antigen-specific antibodies from immunized mice was measured [39] . EAE was induced by subcutaneous injection of mice with 100 μg of myelin oligodendrocyte glycoprotein (MOG 35–55 ) peptides emulsified in complete Freund’s adjuvant. The mice were also injected intraperitoneally with 200 μg pertussis toxin (List Biological Laboratories) on days 0, 1 and 2. All mice were monitored daily for EAE symptoms and scored as follows: 1, tail paralysis; 2, hind-limb weakness; 3, hind-limb paralysis; 4, hind-limb plus fore-limb paralysis; 5, moribund or dead [40] . Blinding experiments were done in EAE. In the adoptive transfer studies, splenic CD4 + T cells (1 × 10 7 cells per mouse) were isolated from donor mice and intravenously transferred into irradiated (5.5 Gy) recipient mice. One day later, the recipient mice were subjected to EAE induction. In addition, the encephalitogenic CD4 + T cells from EAE-diseased mice were isolated and restimulated with MOG (50 μg ml −1 ) in vitro . After 3 days, the encephalitogenic T cells (1 × 10 7 cells per mouse) were intravenously transferred into irradiated (5.5 Gy) recipient mice [41] . The brains and the spinal cords were collected, and infiltrating cells were isolated using Ficoll-Paque PLUS (GE Healthcare). Activation of antigen-specific T cells To determine the activation of antigen-specific T cells, mice were immunized subcutaneously at the tail base with NP–KLH emulsified in aluminium hydroxide gel. T cells that were prepared from the enlarged draining lymph nodes of immunized mice were restimulated with NP–KLH in vitro [39] . Splenocytes and purified T cells from MOG-immunized mice were restimulated with MOG. These T cells were cultured and subjected to cell proliferation and cytokine production analyses [42] . For T-cell proliferation, the restimulated cells were labelled with 1 μCi per well [ 3 H]thymidine and then measured with a scintillation counter. The cytokines in supernatants were collected at 48 h and then were measured by ELISAs. Densitometry and statistical analysis Densitometric analysis of the immunoblotting results was performed using GelPro software (Media Cybernetics). The adequate sample size was determined by the power calculations using G*Power 3.1.6 software. Achieved powers at individual animal experiments were all higher than 0.9. Two-tailed unpaired Student’s t- test and Kruskal–Wallis test were used for statistical analyses. A P -value of less than 0.05 was considered statistically significant. How to cite this article: Li, J.-P. et al . The phosphatase JKAP/DUSP22 inhibits T-cell receptor signalling and autoimmunity by inactivating Lck. Nat. Commun. 5:3618 doi: 10.1038/ncomms4618 (2014).